Prothymosin α overexpression contributes to the development of pulmonary emphysema Emphysema is one of the disease conditions that comprise chronic obstructive pulmonary disease. Prothymosin α transgenic mice exhibit an emphysema phenotype, but the pathophysiological role of prothymosin α in emphysema remains unclear. Here we show that prothymosin α contributes to the pathogenesis of emphysema by increasing acetylation of histones and nuclear factor-kappaB, particularly upon cigarette smoke exposure. We find a positive correlation between prothymosin α levels and the severity of emphysema in prothymosin α transgenic mice and emphysema patients. Prothymosin α overexpression increases susceptibility to cigarette smoke-induced emphysema, and cigarette smoke exposure further enhances prothymosin α expression. We show that prothymosin α inhibits the association of histone deacetylases with histones and nuclear factor-kappaB, and that prothymosin α overexpression increases expression of nuclear factor-kappaB-dependent matrix metalloproteinase 2 and matrix metalloproteinase 9, which are found in the lungs of patients with chronic obstructive pulmonary disease. These results demonstrate the clinical relevance of prothymosin α in regulating acetylation events during the pathogenesis of emphysema. Emphysema, the major consequence of chronic obstructive pulmonary disease (COPD), is characterized by permanent airflow restriction resulting from enlargement of alveolar airspace and loss of lung elasticity [1] . Cigarette smoking is associated with the severity of emphysema, which also correlates with the degree of progressive pulmonary inflammation [2] . Although cigarette smoking is the main risk factor, only about 25% of smokers develop emphysema [3] . Therefore, there may be unidentified genetic or host factors that predispose individuals to emphysema. Prothymosin α (ProT) is a highly acidic nuclear protein, the sequence of which is highly conserved from unicellular organisms to humans; this implies its essential role in cell function [4] , [5] . ProT possesses diverse intracellular and extracellular functions that are involved in proliferation, apoptosis, oxidative stress, immunomodulation and acetylation [6] , [7] , [8] , [9] , [10] , [11] . ProT can bind to the linker histone H1 (refs. 12 , 13 ) and core histones [14] , thereby modulating the chromatin structure. As chromatin remodelling is regulated by the acetylation and deacetylation of histones, recent studies have explored the acetylation-regulating role of ProT. ProT can interact with two different histone acetyltransferases (HATs): CREB-binding protein (CBP) and p300 (refs. 15 , 16 ). ProT stimulates AP1- and NF-κB-dependent transcription through interaction with CBP [17] . Moreover, overexpression of ProT elicits a p53 response that involves p53 acetylation [18] . Although ProT appears to be involved in multiple cellular functions, its exact physiological role remains poorly understood. We have generated ProT transgenic mice that exhibit the polycystic kidney disease phenotype, which is characterized by the development of renal cysts and progressive renal dysfunction [19] , as well as emphysema-like changes in the lung. However, the pathophysiological role of ProT in pulmonary emphysema remains unknown. The aim of this study was to gain insight into the molecular mechanisms underlying the action of ProT on the development of emphysema, particularly under the stimulation of cigarette smoke (CS). Our results from animal models and clinical patients support an important role for ProT in the development of emphysema. We show that ProT can enhance the acetylation of histones and nuclear factor-kappaB (NF-κB), leading to activating NF-κB and upregulating NF-κB-dependent pro-inflammatory gene expression, including matrix metalloproteinase 2 (MMP2) and matrix metalloproteinase 9 (MMP9). Our findings elucidate the pathophysiological role of ProT and identify a potential novel molecular mechanism in the pathogenesis of COPD. ProT overexpression leads to an emphysema-like phenotype ProT homozygous (HZ) transgenic mice spontaneously developed pulmonary emphysema characterized by alveolar airspace enlargement and alveolar wall destruction, whereas heterozygous (HET) mice had only mild disease ( Fig. 1a , left). The average airspace in the HZ mice was four-fold greater than that in the non-transgenic (NT) littermates ( Fig. 1b , right). HZ mice died at 10 days postpartum, whereas heterozygotes appeared normal and lived their normal life span [19] . The overexpression of ProT was confirmed immunohistochemically in the emphysematous tissues of the transgenic mice ( Fig. 1b ). There was a positive correlation between ProT levels and the severity of emphysema, as assessed by airspace enlargement ( Fig. 1c ). 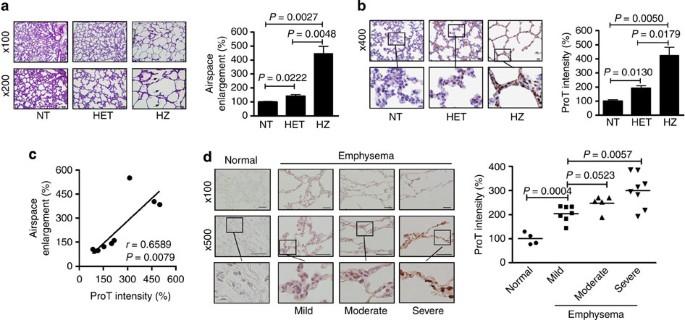Figure 1: Overexpression of ProT in transgenic mice and in the lung epithelium of patients with emphysema. (a) H&E-stained lung sections of 4-day-old ProT HZ, HET and NT mice (left) and quantitative analysis of alveolar airspace enlargement (right). Scale bars shown on × 100 and × 200 images correspond to 100 and 50 μm, respectively. Average airspace area was calculated by dividing the total airspace by the total number of alveoli in three randomly selected fields at × 200 magnification in each section. Values (mean±s.e.m.,n=3; Student’st-test) shown are relative airspace area, with the value of NT mice arbitrarily set to 100. Arrow denotes alveolar wall destruction. (b) Immunohistochemistry (left) and quantitation (right) of ProT in the lung sections of mice. Its immunoreactive intensity (mean±s.e.m.,n=3; Student’st-test) was analysed by MetaMorph software. Scale bars shown on × 400 images correspond to 20 μm, and the boxed areas are magnified below each panel. (c) A positive correlation (P=0.0079; Pearson’s correlation coefficient) between the levels of ProT immunoreactivity and airspace enlargement. (d) Immunohistochemistry (right) and quantitation (left) of ProT in lung tissues from patients with emphysema of varying severity and non-COPD individuals. Scale bars shown on × 100 and × 500 images correspond to 200 and 100 μm, respectively, and the boxed areas are magnified below each panel. Values shown are levels of ProT immunoreactivity in individual specimens, with the mean level in normal tissues arbitrarily set to 100, in three randomly selected fields at × 500 magnification in each section; horizontal bars represent the mean (n=4–8; Student’st-test). Results are representative of three independent experiments. Figure 1: Overexpression of ProT in transgenic mice and in the lung epithelium of patients with emphysema. ( a ) H&E-stained lung sections of 4-day-old ProT HZ, HET and NT mice (left) and quantitative analysis of alveolar airspace enlargement (right). Scale bars shown on × 100 and × 200 images correspond to 100 and 50 μm, respectively. Average airspace area was calculated by dividing the total airspace by the total number of alveoli in three randomly selected fields at × 200 magnification in each section. Values (mean±s.e.m., n =3; Student’s t -test) shown are relative airspace area, with the value of NT mice arbitrarily set to 100. Arrow denotes alveolar wall destruction. ( b ) Immunohistochemistry (left) and quantitation (right) of ProT in the lung sections of mice. Its immunoreactive intensity (mean±s.e.m., n =3; Student’s t -test) was analysed by MetaMorph software. Scale bars shown on × 400 images correspond to 20 μm, and the boxed areas are magnified below each panel. ( c ) A positive correlation ( P =0.0079; Pearson’s correlation coefficient) between the levels of ProT immunoreactivity and airspace enlargement. ( d ) Immunohistochemistry (right) and quantitation (left) of ProT in lung tissues from patients with emphysema of varying severity and non-COPD individuals. Scale bars shown on × 100 and × 500 images correspond to 200 and 100 μm, respectively, and the boxed areas are magnified below each panel. Values shown are levels of ProT immunoreactivity in individual specimens, with the mean level in normal tissues arbitrarily set to 100, in three randomly selected fields at × 500 magnification in each section; horizontal bars represent the mean ( n =4–8; Student’s t -test). Results are representative of three independent experiments. Full size image ProT is overexpressed in the lung of emphysema patients To further explore whether emphysema induced by ProT overexpression in transgenic mice resembled human emphysema, we examined 20 clinical specimens from patients with varying degrees of pulmonary emphysema—15 smokers and 5 non-smokers—for ProT expression ( Supplementary Table S1 ). The patients had been diagnosed with emphysema on the basis of pulmonary function test results, computed tomography (CT) scans and pathological reports from resected lung specimens. Overall, ProT was overexpressed in 19 (95%) of the 20 emphysematous specimens. However, it was expressed only weakly in four non-tumourous, normal lung tissues obtained from lung cancer patients who were cigarette smokers without COPD ( Fig. 1d , left, Supplementary Fig. S1a,b , Supplementary Table S1 ). These results further support the involvement of ProT in emphysema. Notably, with regard to the intensity of ProT immunoreactivity, the degree of ProT expression was positively correlated with the severity of emphysema in the patients ( Fig. 1d , right, Supplementary Table S1 ). ProT transgenic mice are susceptible to CS-induced emphysema Given that CS is the main risk factor for emphysema, we next investigated whether treatment with CS extract (CSE) resulted in overexpression of ProT. We analysed the microarray data [20] (Gene Expression Omnibus (GEO) accession number GPL96 , Data Set Record GDS737) obtained from the GEO, NCBI and found that smokers with severe emphysema had significantly higher levels of ProT expression in the lungs than smokers with mild or no emphysema ( Supplementary Fig. S2 ). These data suggest that ProT may predispose individuals to CS-induced emphysema. We further investigated this issue using a mouse model of emphysema induced by CSE. We successfully established an emphysema model using wild-type FVB mice treated with CSE for 5 to 7 weeks ( Supplementary Fig. S3 ). We demonstrated that, like rats, as previously reported [21] , mice can serve as a useful animal model of CSE-induced emphysema that closely resembles the form produced in rats and is similar to that found in humans. To determine the role of ProT in the susceptibility of mice to CSE-induced emphysema, we exposed ProT HET and NT mice to CSE and examined their lungs for airspace enlargement. Immunohistochemical examination ( Fig. 2a , left) and quantification of the immunoreactive intensity ( Fig. 2a , right) confirmed that the ProT levels in ProT transgenic mice were higher than in NT mice and increased further after CSE treatment ( Fig. 2a , right). As shown in Fig. 2b (left), 27% of the ProT transgenic mice spontaneously developed emphysema, whereas none of the NT mice developed the disease. However, treatment with CSE dramatically increased the incidence of emphysema, with 100% of ProT heterozygotes and 67% of NT mice exhibiting airspace enlargement. Furthermore, the transgenic mice had more severe disease than the NT mice after CSE treatment ( Fig. 2b , middle, right). To further support the physiological association of ProT with the development of emphysema, we delivered lentiviral vectors expressing ProT short hairpin RNA (shRNA) into the lungs of wild-type FVB mice to knockdown the endogenous ProT expression ( Fig. 2c , left, right). This resulted in concomitant decreases in the incidence ( Fig. 2d , left) and severity ( Fig. 2d , middle, right) of emphysema after CSE treatment. Collectively, these results highlight the importance of ProT in the development of emphysema and further suggest that overexpressed ProT in the lung may increase susceptibility to emphysema either related or unrelated to CS exposure. 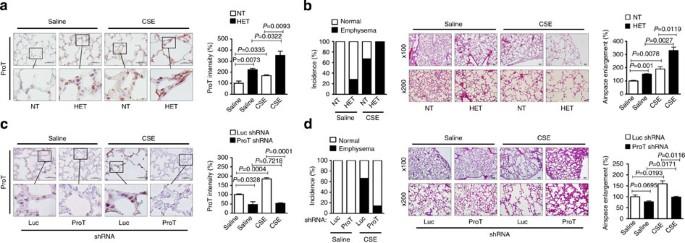Figure 2: ProT is involved in CSE-induced emphysema in mice. (a,b) Six-week-old ProT HET and NT mice were injected intraperitoneally with CSE or saline twice a week for 6 weeks. (c,d) Six-week-old FVB mice were intratracheally injected with lentiviral vectors expressing ProT or luciferase (Luc) shRNA followed by intraperitoneal injections of CSE or saline twice a week for 6 weeks. Subsequently, their lung sections were immunostained for ProT (a,c) and H&E stained for examining alveolar airspace enlargement (b,d), as described inFigure 1. The boxed areas in upper panels (original magnification × 400; Scale bar=100 μm) are magnified and shown in lower panels (a,c) and scale bars on × 100 and × 200 images correspond to 100 and 50 μm, respectively (b,d). Histological changes in the lungs were evaluated for the incidence of emphysema in ProT transgenic or NT mice (0 of 13 for NT-Saline, 3 of 11 for HET-Saline, 10 of 15 for NT-CSE and 10 of 10 for HET-CSE;P<0.0001 between any two of the four treatment groups analysed by theχ2-test) (b), and in ProT knockdown mice (0 of 6 for Luc shRNA-Saline, 0 of 6 for ProT shRNA-Saline, 6 of 9 Luc shRNA-CSE and 1 of 7 ProT shRNA-CSE;P<0.0001 between any two of the four treatment groups analysed by theχ2-test) (d). All immunohistochemical and histochemical data (mean±s.e.m.,n=3; Student’st-test) are representative of three independent experiments. Figure 2: ProT is involved in CSE-induced emphysema in mice. ( a , b ) Six-week-old ProT HET and NT mice were injected intraperitoneally with CSE or saline twice a week for 6 weeks. ( c , d ) Six-week-old FVB mice were intratracheally injected with lentiviral vectors expressing ProT or luciferase (Luc) shRNA followed by intraperitoneal injections of CSE or saline twice a week for 6 weeks. Subsequently, their lung sections were immunostained for ProT ( a , c ) and H&E stained for examining alveolar airspace enlargement ( b , d ), as described in Figure 1 . The boxed areas in upper panels (original magnification × 400; Scale bar=100 μm) are magnified and shown in lower panels ( a , c ) and scale bars on × 100 and × 200 images correspond to 100 and 50 μm, respectively ( b , d ). Histological changes in the lungs were evaluated for the incidence of emphysema in ProT transgenic or NT mice (0 of 13 for NT-Saline, 3 of 11 for HET-Saline, 10 of 15 for NT-CSE and 10 of 10 for HET-CSE; P <0.0001 between any two of the four treatment groups analysed by the χ 2 -test) ( b ), and in ProT knockdown mice (0 of 6 for Luc shRNA-Saline, 0 of 6 for ProT shRNA-Saline, 6 of 9 Luc shRNA-CSE and 1 of 7 ProT shRNA-CSE; P <0.0001 between any two of the four treatment groups analysed by the χ 2 -test) ( d ). All immunohistochemical and histochemical data (mean±s.e.m., n =3; Student’s t -test) are representative of three independent experiments. Full size image ProT inhibits histone deacetylases Given the decreased histone deacetylases (HDAC) activity in the peripheral lungs and alveolar macrophages in COPD patients, and the resulting amplification of pro-inflammatory gene expression through increased histone acetylation [2] , [22] , we investigated whether HDACs were affected in the lungs of emphysema patients and ProT transgenic mice. Immunohistochemical examination revealed lower levels of HDAC2 expression in the lung epithelia of patients with more severe emphysema, despite little change in HDAC1 and HDAC3 levels ( Fig. 3a ). Similar expression patterns of HDACs were noted in ProT transgenic mice, particularly in the homozygotes, as detected by immunohistochemistry ( Fig. 3b ) and immunoblotting ( Fig. 3c ). 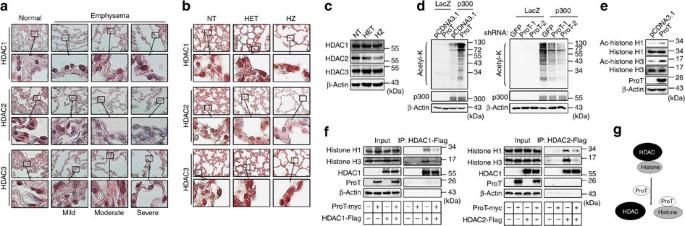Figure 3: Overexpression of ProT inhibits HDACs and enhances protein acetylation. (a,b) Immunohistochemical staining for HDACs. Lung tissues from patients with emphysema of varying severity and non-COPD individuals (a), as well as lung tissues from 4-day-old ProT HZ, HET and NT mice (b) were immunostained with monoclonal antibody against HDAC1, HDAC2 and HDAC3. Note that lower levels of HDAC2, but not HDAC1 and HDAC3, were detected in patients with more severe emphysema and in ProT HZ mice, as compared with their normal counterparts. The boxed areas in upper panels (original magnification × 400; scale bar=100 μm) are magnified and shown in lower panels. (c) Immunoblot analysis of HDACs in the lung tissues of 4-day-old ProT HZ, HET and NT mice. (d) Detection of acetylated-lysine (acetyl-K). 293T cells that had been transfected with pcDNA3.1-ProT-myc/His or pcDNA3.1 (left) or transduced with lentiviral vectors expressing ProT shRNA-1 and -2 or GFP shRNA (right) were transfected with a p300 expression plasmid (pCMVb p300 HA tag) or a control plasmid (pHM6-lacZ). After 24 h, total cell lysates were examined for the indicated proteins by immunoblotting. Equal levels of p300 and LacZ expression were verified. (e) Detection of acetylated histones. 293 T cells were transfected with pcDNA3.1-ProT-myc/His or pcDNA3.1 and their total cell lysates were examined for the indicated proteins by immunoblotting after 24 h. (f) HDAC and histone binding assay. 293T cells that had been transduced with HDAC1-Flag (pcDNA3.1-HDAC1-Flag) (left) or HDAC2-Flag (pCMV-Tag4C-HDAC2) (right) were transfected with pcDNA3.1-ProT-myc/His or pcDNA3.1. Total cell lysates were immunoprecipitated by Flag-M2 beads and analysed by immunoblotting for the indicated proteins. Whole-cell lysates without immunoprecipitation (10% input) were estimated for the expression levels of histone H1 and H3, HDAC1, HDAC2 and ProT by immunoblotting. (g) Proposed model for ProT-mediated enhancement of histone acetylation via HDAC/histone dissociation. Results are representative of three independent experiments. Figure 3: Overexpression of ProT inhibits HDACs and enhances protein acetylation. ( a , b ) Immunohistochemical staining for HDACs. Lung tissues from patients with emphysema of varying severity and non-COPD individuals ( a ), as well as lung tissues from 4-day-old ProT HZ, HET and NT mice ( b ) were immunostained with monoclonal antibody against HDAC1, HDAC2 and HDAC3. Note that lower levels of HDAC2, but not HDAC1 and HDAC3, were detected in patients with more severe emphysema and in ProT HZ mice, as compared with their normal counterparts. The boxed areas in upper panels (original magnification × 400; scale bar=100 μm) are magnified and shown in lower panels. ( c ) Immunoblot analysis of HDACs in the lung tissues of 4-day-old ProT HZ, HET and NT mice. ( d ) Detection of acetylated-lysine (acetyl-K). 293T cells that had been transfected with pcDNA3.1-ProT-myc/His or pcDNA3.1 (left) or transduced with lentiviral vectors expressing ProT shRNA-1 and -2 or GFP shRNA (right) were transfected with a p300 expression plasmid (pCMVb p300 HA tag) or a control plasmid (pHM6-lacZ). After 24 h, total cell lysates were examined for the indicated proteins by immunoblotting. Equal levels of p300 and LacZ expression were verified. ( e ) Detection of acetylated histones. 293 T cells were transfected with pcDNA3.1-ProT-myc/His or pcDNA3.1 and their total cell lysates were examined for the indicated proteins by immunoblotting after 24 h. ( f ) HDAC and histone binding assay. 293T cells that had been transduced with HDAC1-Flag (pcDNA3.1-HDAC1-Flag) (left) or HDAC2-Flag (pCMV-Tag4C-HDAC2) (right) were transfected with pcDNA3.1-ProT-myc/His or pcDNA3.1. Total cell lysates were immunoprecipitated by Flag-M2 beads and analysed by immunoblotting for the indicated proteins. Whole-cell lysates without immunoprecipitation (10% input) were estimated for the expression levels of histone H1 and H3, HDAC1, HDAC2 and ProT by immunoblotting. ( g ) Proposed model for ProT-mediated enhancement of histone acetylation via HDAC/histone dissociation. Results are representative of three independent experiments. Full size image As ProT can interact with histones [12] , [13] , [14] and CBP/p300 (refs. 15 , 16 ), it may affect chromatin remodelling processes and regulate transcription. Overexpressed ProT has been shown to elicit a p53 response that involves acetylation of p53 at residues known to be acetylated by CBP/p300 (ref. 12 ). We hypothesized that ProT may be involved in the regulation of protein acetylation that contributes to the development of emphysema. We used overexpression and knockdown experiments to study whether ProT could mediate protein acetylation. E1A and SV40 large T antigen, which are constitutively expressed in 293 T cells, can bind CBP/p300 and reduce the amount of active CBP/p300 (refs. 23 , 24 ). Therefore, the p300 deletion mutant lacking the CH3 interaction domain (missing amino acids 1737–1836) was employed for transfection to 293T cells given its well-defined inability to interact with E1A and SV40 large T antigen. In p300-overexpressing 293T cells, overexpressed ProT dramatically increased lysine acetylation in a large number of proteins ( Fig. 3d , left), whereas knockdown of endogenous ProT dramatically suppressed acetylation events ( Fig. 3d , right). These findings suggest that ProT may have a global role in protein acetylation. We further showed that overexpression of ProT not only enhanced the acetylation of histone H1 and H3 ( Fig. 3e ), but also decreased the association of HDAC1 ( Fig. 3f , left) and HDAC2 ( Fig. 3f , right) with histones H1 and H3. These results suggest that ProT may enhance protein acetylation by inhibiting the binding of HDACs to histones ( Fig. 3g ). ProT increases protein acetylation in the emphysematous lung We further investigated whether ProT-mediated increases in protein acetylation found in cultured cells could also be detected in ProT transgenic mice and emphysema patients. The intracellular levels of acetylated-lysine (acetyl-K) in the lung epithelium were significantly higher in homozygotes than in heterozygotes ( Fig. 4a ). Furthermore, there was a positive correlation between the levels of ProT and those of acetyl-K in the transgenic mice ( Fig. 4b ). With the exception of two clinical specimens of mild emphysema that showed single-positive staining for either ProT or acetyl-K, 18 of the 20 clinical specimens of emphysema were found to be immunoreactive for both ProT and acetyl-K ( Fig. 4c , Supplementary Figs 1a,1b,4a,4b ). Notably, higher levels of acetylation were visualized in the nuclei of cells from patients with severe emphysema ( Fig. 4c , upper). Quantification of the immunoreactive intensity revealed higher acetyl-K levels in patients with more severe emphysema than in those with mild emphysema ( Fig. 4c , lower). Immunofluorescence staining demonstrated nuclear colocalization of acetyl-K with ProT in the specimens from patients with severe emphysema ( Fig. 4d ). This suggests that ProT is involved in lysine acetylation events. Furthermore, there was a positive correlation between the expression levels of ProT and those of acetyl-K in the clinical specimens ( Fig. 4e ). ProT HET mice showed higher levels of acetyl-K compared with NT littermates, which were further increased after CSE treatment ( Fig. 4f ). 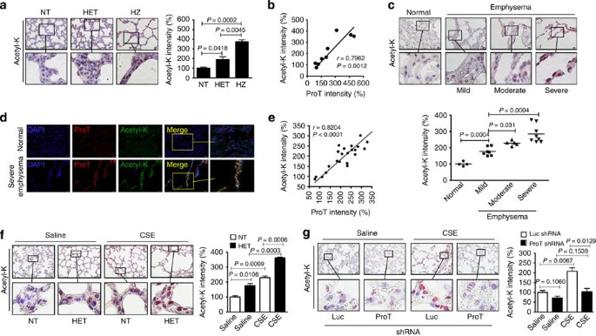Figure 4: Overexpression of ProT increases protein acetylation in emphysematous lungs of mice and patients. (a) Immunohistochemistry (left) and quantitation (right) of acetylated-lysine (acetyl-K) in lung tissues of 4-day-old ProT HZ, HET and NT mice. (b) A positive correlation (P=0.0012; Pearson’s correlation coefficient) between the levels of ProT immunoreactivity and those of acetylated-lysine immunoreactivity. (c) Immunohistochemistry (upper) and quantitation (lower) of acetyl-K in lung tissues from patients with emphysema of varying severity and non-COPD individuals. Values shown are immunoreactive levels in individual specimens; horizontal bars represent the mean. (d) Immunofluorescence microscopy. Lung tissues from patients with severe emphysema and from non-COPD individuals were incubated with mouse monoclonal antibody against ProT and rabbit polyclonal antibody against acetyl-K followed by Alexa Fluor 594-conjugated goat anti-mouse IgG and FITC-conjugated goat anti-rabbit IgG. Nuclei were counterstained with DAPI. Fluorescence signals for ProT (red), acetyl-K (green) and the nucleus (blue) were examined by fluorescence microscopy. (e) A positive correlation (P<0.0001; Pearson’s correlation coefficient) between the levels of ProT immunoreactivity and those of acetyl-K immunoreactivity. (f,g) Immunohistochemistry (left) and quantitation (right) of acetyl-K in lung tissues from ProT HET and NT mice that were injected intraperitoneally with CSE or saline twice a week for 6 weeks (f) and from FVB mice that had been intratracheally injected with lentiviral vectors expressing ProT or luciferase (Luc) shRNA followed by intraperitoneal injections of CSE or saline twice a week for 6 weeks (g). Acetyl-K immunoreactive intensity (mean±s.e.m.; Student’st-test) was analysed in three randomly selected fields at × 400 magnification in each section by MetaMorph software (n=3 in (a,f,g);n=4–8 inc). Values shown are relative acetyl-K intensity levels, with the level in normal tissues arbitrarily set to 100. Scale bar=20 μm, and the boxed areas in upper panels (original magnification × 400) are magnified and shown in lower panels. Results are representative of three independent experiments. Figure 4: Overexpression of ProT increases protein acetylation in emphysematous lungs of mice and patients. ( a ) Immunohistochemistry (left) and quantitation (right) of acetylated-lysine (acetyl-K) in lung tissues of 4-day-old ProT HZ, HET and NT mice. ( b ) A positive correlation ( P =0.0012; Pearson’s correlation coefficient) between the levels of ProT immunoreactivity and those of acetylated-lysine immunoreactivity. ( c ) Immunohistochemistry (upper) and quantitation (lower) of acetyl-K in lung tissues from patients with emphysema of varying severity and non-COPD individuals. Values shown are immunoreactive levels in individual specimens; horizontal bars represent the mean. ( d ) Immunofluorescence microscopy. Lung tissues from patients with severe emphysema and from non-COPD individuals were incubated with mouse monoclonal antibody against ProT and rabbit polyclonal antibody against acetyl-K followed by Alexa Fluor 594-conjugated goat anti-mouse IgG and FITC-conjugated goat anti-rabbit IgG. Nuclei were counterstained with DAPI. Fluorescence signals for ProT (red), acetyl-K (green) and the nucleus (blue) were examined by fluorescence microscopy. ( e ) A positive correlation ( P <0.0001; Pearson’s correlation coefficient) between the levels of ProT immunoreactivity and those of acetyl-K immunoreactivity. ( f , g ) Immunohistochemistry (left) and quantitation (right) of acetyl-K in lung tissues from ProT HET and NT mice that were injected intraperitoneally with CSE or saline twice a week for 6 weeks ( f ) and from FVB mice that had been intratracheally injected with lentiviral vectors expressing ProT or luciferase (Luc) shRNA followed by intraperitoneal injections of CSE or saline twice a week for 6 weeks ( g ). Acetyl-K immunoreactive intensity (mean±s.e.m. ; Student’s t -test) was analysed in three randomly selected fields at × 400 magnification in each section by MetaMorph software ( n =3 in ( a , f , g ); n =4–8 in c ). Values shown are relative acetyl-K intensity levels, with the level in normal tissues arbitrarily set to 100. Scale bar=20 μm, and the boxed areas in upper panels (original magnification × 400) are magnified and shown in lower panels. Results are representative of three independent experiments. Full size image To further verify the physiological importance of ProT in the CSE-induced enhancement of acetylation events, we knocked down endogenous ProT in the mouse lung. Results from immunohistochemistry ( Fig. 4g , left) and quantitative analysis ( Fig. 4g , right) revealed that suppression of endogenous ProT resulted in the attenuation of CSE-induced enhancement of acetyl-K levels. Notably, a higher degree of lysine acetylation corresponded to a more severe enlargement of alveolar airspace ( Fig. 4f ). Collectively, these results strongly indicate the involvement of ProT in regulating protein acetylation in emphysema in general and in CS-mediated emphysema in particular. ProT regulates NF-κB acetylation in emphysema Given that ProT can regulate the transcriptional activity of NF-κB through interaction with CBP [17] and that activity of NF-κB is post-translationally regulated by HAT-mediated acetylation and repressed by HDACs, especially HDAC3 (refs. 25 ), we next explored whether ProT has a role in regulating NF-κB acetylation in emphysema. Overexpression of ProT increased acetylation of NF-κB RelA/p65 subunit at Lys310, which is required for its full transactivation function [26] ( Fig. 5a , left) and the transcriptional activity of NF-κB (5b, left), whereas knockdown of endogenous ProT abolished such effects ( Fig. 5a , right, Fig. 5b , right). Moreover, the direct interaction of endogenous p65 with ProT was verified in 293T cells overexpressing ProT ( Fig. 5c ). As ProT could regulate histone acetylation by inhibiting the association of HDACs with histones ( Fig. 3f ), we next examined whether the ProT-mediated enhancement of NF-κB acetylation could be ascribed to the same mechanism. Immunoprecipitation with anti-Flag antibody and immunoblotting with HDAC3 antibody of 293T cells cotransfected with ProT-myc/His vector and NF-κB p65-Flag vector revealed that overexpression of ProT reduced the interaction of NF-κB with HDAC3, as a lower amount of HDAC3 was pulled down along with p65 in ProT-overexpressing cells compared with the corresponding control cells ( Fig. 5d , left). In reverse immunoprecipitation, similar results were obtained in cells cotransfected with ProT-myc/His vector and HDAC3-Flag vector, showing that a lower amount of p65 was pulled down along with HDAC3 ( Fig. 5d , right). As ProT could interact with p65 ( Fig. 5c ) and enhance its acetylation ( Fig. 5a ), we further investigated whether ProT could affect the interaction of p300 with NF-κB. 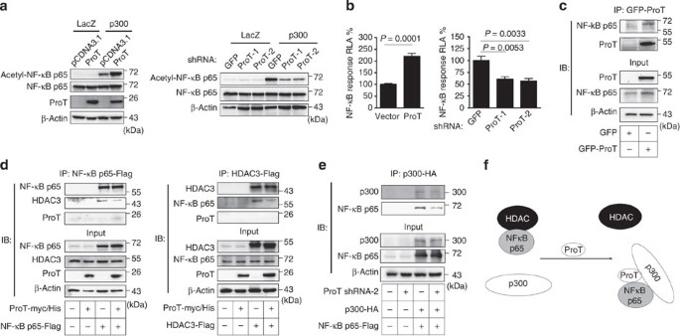Figure 5: Overexpression of ProT increases NF-κB acetylation. (a) Detection of acetylated NF-κB p65 (Lys310). 293T cells that had been transfected with pcDNA3.1-ProT-myc/His or pcDNA3.1 (left) or transduced with lentiviruses expressing ProT shRNA-1 and -2 or GFP shRNA (right) were transfected with a p300 expression vector (pCMVb p300 HA delta33) or a control vector (pHM6-lacZ). After 24 h, total cell lysates were examined for the indicated proteins by immunoblotting. Equal levels of p300 and LacZ expression in the transfected cells were verified. (b) Reporter assay for NF-κB transactivation activity. 293T cells that had been transduced with lentiviruses expressing ProT-IRES-GFP or GFP alone (left), or ProT or GFP shRNA (right) were cotransfected with pNF-κB-Luc and pTK-Renilla reporter plasmids. Total cell lysates were harvested 48 h later, and their firefly andRenillaluciferase activities were determined. The ratio of firefly luciferase activity toRenillaluciferase activity was expressed as relative light activity. Values shown are the mean±s.e.m. (n=4 for left andn=5 for right; Student’st-test). (c) NF-κB and ProT binding assay. Cell lysates from 293T cells transduced with lentiviruses expressing GFP-tagged ProT or GFP alone were immuoprecipitated by anti-GFP monoclonal antibody followed by immunoblotting with anti-NF-κB p65 and anti-GFP antibody. Whole-cell lysates without immunoprecipitation (10% input) were estimated for the expression levels of NF-κB and ProT by immunoblotting. (d) Analysis of the effect of ProT on NF-κB and HDAC3 binding. 293T cells that had been transfected with an NF-κB p65 expression vector (pcDNA3-cFlag-RelA) or a control vector (pCMV-Tag2B) (left) or HDAC3 expression vector (pcDNA3.1-HDAC3-Flag) or a control vector (pCMV-Tag2B) (right) were transfected with pcDNA3.1-ProT-myc/His or pcDNA3.1. After 24 h, total cell lysates were immuoprecipitated by Flag-M2 beads followed by immunoblotting with the indicated proteins. Whole-cell lysates without immunoprecipitation (10% input) were estimated by immunoblotting with indicated proteins. (e) p300 and NF-κB binding assay. 293T cells that had been transduced with lentiviruses expressing ProT shRNA-2 or luciferase shRNA as the control were transfected with the pCMVb p300 HA delta33 and pcDNA3-cFlag-RelA. Total cell lysates were immunoprecipitated by anti-HA antibody followed by immunoblotting with the indicated proteins. Results are representative of three independent experiments. (f) Proposed model for ProT-mediated NF-κB hyperacetylation via HDAC3/NF-κB dissociation and p300/NF-κB association. Figure 5e shows that knockdown of endogenous ProT attenuated the interaction of p300 with NF-κB, as a lower amount of p65 was pulled down along with p300 in ProT knockdown cells that had been cotransfected with p300 HA and NF-κB p65-Flag vectors. Collectively, these results indicate that ProT can increase NF-κB acetylation both by depriving HDACs from NF-κB and by facilitating the recruitment of p300 to NF-κB ( Fig. 5f ). Figure 5: Overexpression of ProT increases NF-κB acetylation. ( a ) Detection of acetylated NF-κB p65 (Lys310). 293T cells that had been transfected with pcDNA3.1-ProT-myc/His or pcDNA3.1 (left) or transduced with lentiviruses expressing ProT shRNA-1 and -2 or GFP shRNA (right) were transfected with a p300 expression vector (pCMVb p300 HA delta33) or a control vector (pHM6-lacZ). After 24 h, total cell lysates were examined for the indicated proteins by immunoblotting. Equal levels of p300 and LacZ expression in the transfected cells were verified. ( b ) Reporter assay for NF-κB transactivation activity. 293T cells that had been transduced with lentiviruses expressing ProT-IRES-GFP or GFP alone (left), or ProT or GFP shRNA (right) were cotransfected with pNF-κB-Luc and pTK-Renilla reporter plasmids. Total cell lysates were harvested 48 h later, and their firefly and Renilla luciferase activities were determined. The ratio of firefly luciferase activity to Renilla luciferase activity was expressed as relative light activity. Values shown are the mean±s.e.m. ( n =4 for left and n =5 for right; Student’s t -test). ( c ) NF-κB and ProT binding assay. Cell lysates from 293T cells transduced with lentiviruses expressing GFP-tagged ProT or GFP alone were immuoprecipitated by anti-GFP monoclonal antibody followed by immunoblotting with anti-NF-κB p65 and anti-GFP antibody. Whole-cell lysates without immunoprecipitation (10% input) were estimated for the expression levels of NF-κB and ProT by immunoblotting. ( d ) Analysis of the effect of ProT on NF-κB and HDAC3 binding. 293T cells that had been transfected with an NF-κB p65 expression vector (pcDNA3-cFlag-RelA) or a control vector (pCMV-Tag2B) (left) or HDAC3 expression vector (pcDNA3.1-HDAC3-Flag) or a control vector (pCMV-Tag2B) (right) were transfected with pcDNA3.1-ProT-myc/His or pcDNA3.1. After 24 h, total cell lysates were immuoprecipitated by Flag-M2 beads followed by immunoblotting with the indicated proteins. Whole-cell lysates without immunoprecipitation (10% input) were estimated by immunoblotting with indicated proteins. ( e ) p300 and NF-κB binding assay. 293T cells that had been transduced with lentiviruses expressing ProT shRNA-2 or luciferase shRNA as the control were transfected with the pCMVb p300 HA delta33 and pcDNA3-cFlag-RelA. Total cell lysates were immunoprecipitated by anti-HA antibody followed by immunoblotting with the indicated proteins. Results are representative of three independent experiments. ( f ) Proposed model for ProT-mediated NF-κB hyperacetylation via HDAC3/NF-κB dissociation and p300/NF-κB association. Full size image We further investigated whether ProT-mediated NF-κB acetylation at Lys310 was associated with emphysema. Increased acetyl-NF-κB expression was detected in the lung epithelia of ProT transgenic mice, in particular in the homozygotes ( Fig. 6a ), and of patients with emphysema ( Fig. 6b ). Notably, patients with more severe emphysema appeared to have higher levels of acetyl-NF-κB ( Fig. 6b ). The contribution of ProT in mediating NF-κB acetylation in vivo was further verified by ProT knockdown experiments in wild-type FVB mice. The knockdown of endogenous ProT in the lungs via intratracheal administration of lentiviral vectors expressing ProT shRNA reduced CSE-mediated NF-κB acetylation ( Fig. 6c ). Immunofluorescence staining showed that treatment with CSE increased the nuclear translocation of NF-κB, which colocalized with ProT, in the lungs of ProT HET mice ( Fig. 6d ) and in mouse lung epithelial MLE 12 cells transduced with ProT ( Fig. 6e ). Taken together, these results indicate that ProT can regulate the acetylation and activity of NF-κB in emphysematous lungs, which is likely through its dual effect of increasing the association of p300 with NF-κB and decreasing the association of HDACs with NF-κB. 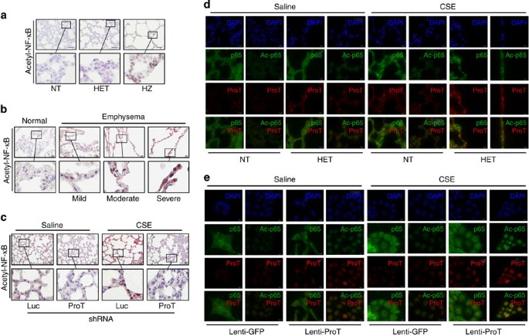Figure 6: Overexpression of ProT increases NF-κB acetylation in emphysematous lungs of mice and patients. (a–c) Immunohistochemical detection of acetyl-NF-κB p65 in lung tissues from 4-day-old ProT HZ, HET and NT mice (a), from patients with emphysema of varying severity and non-COPD individuals (b) and from FVB mice that had been intratracheally injected with lentiviral vectors expressing ProT or luciferase (Luc) shRNA followed by intraperitoneal injections of CSE or saline twice a week for 6 weeks (c). Note that positive nuclear staining for acetyl-NF-κB p65 in the lung epithelium of ProT transgenic mice was observed (a) and that higher levels of acetyl-NF-κB p65 accumulation were detected in patients with more severe emphysema (b). The boxed areas in upper panels (original magnification × 400; Scale bar=20 μm) are magnified and shown in lower panels. (d,e) Immunofluorescence microscopy. Lung tissues from ProT HET and NT mice that had been injected intraperitoneally with CSE or saline twice a week for 6 weeks (d) and mouse lung epithelial MLE 12 cells that had been transduced with ProT and GFP by lentiviral vectors Lenti-ProT and Lenti-GFP, respectively, and then treated with CSE or saline (e) were incubated with mouse monoclonal antibody against ProT and rabbit polyclonal antibody against NF-κB p65 or acetyl-NF-κB p65 (Lys310) followed by Alexa Fluor 594-conjugated goat anti-mouse IgG and Alexa Fluor 488-conjugated goat anti-rabbit IgG. Nuclei were counterstained with DAPI. Fluorescence signals for ProT (red), NF-κB p65 (green), acetyl-NF-κB p65 (green) and the nucleus (blue) were examined by fluorescence microscopy. Scale bar=10 μm; original magnification × 400. Results are representative of three independent experiments. Figure 6: Overexpression of ProT increases NF-κB acetylation in emphysematous lungs of mice and patients. ( a – c ) Immunohistochemical detection of acetyl-NF-κB p65 in lung tissues from 4-day-old ProT HZ, HET and NT mice ( a ), from patients with emphysema of varying severity and non-COPD individuals ( b ) and from FVB mice that had been intratracheally injected with lentiviral vectors expressing ProT or luciferase (Luc) shRNA followed by intraperitoneal injections of CSE or saline twice a week for 6 weeks ( c ). Note that positive nuclear staining for acetyl-NF-κB p65 in the lung epithelium of ProT transgenic mice was observed ( a ) and that higher levels of acetyl-NF-κB p65 accumulation were detected in patients with more severe emphysema ( b ). The boxed areas in upper panels (original magnification × 400; Scale bar=20 μm) are magnified and shown in lower panels. ( d , e ) Immunofluorescence microscopy. Lung tissues from ProT HET and NT mice that had been injected intraperitoneally with CSE or saline twice a week for 6 weeks ( d ) and mouse lung epithelial MLE 12 cells that had been transduced with ProT and GFP by lentiviral vectors Lenti-ProT and Lenti-GFP, respectively, and then treated with CSE or saline ( e ) were incubated with mouse monoclonal antibody against ProT and rabbit polyclonal antibody against NF-κB p65 or acetyl-NF-κB p65 (Lys310) followed by Alexa Fluor 594-conjugated goat anti-mouse IgG and Alexa Fluor 488-conjugated goat anti-rabbit IgG. Nuclei were counterstained with DAPI. Fluorescence signals for ProT (red), NF-κB p65 (green), acetyl-NF-κB p65 (green) and the nucleus (blue) were examined by fluorescence microscopy. Scale bar=10 μm; original magnification × 400. Results are representative of three independent experiments. Full size image ProT regulates the production of MMP2 and MMP9 in emphysema Abnormal production of MMPs is implicated in the pathogenesis of emphysema. Human studies have also demonstrated oversecretion of MMP2 and MMP9 in patients with COPD [27] . As the promoter regions of MMP2 and MMP9 contain binding sites for NF-κB and their expression is regulated by NF-κB (refs. 28 , 29 , 30 ), we examined whether the production of MMP2 and MMP9 was regulated by ProT in emphysema. Higher levels of MMP2 and MMP9 proteins were detected in human emphysematous tissues than in normal tissues ( Fig. 7a ). In the mouse lung tissue, ProT transgenic mice exhibited increased expression of MMP2 and MMP9 proteins ( Fig. 7b ) and mRNA ( Fig. 7c ), compared with NT littermates. Gelatin zymography also revealed higher MMP2 and MMP9 activity in the HZ mouse embryonic fibroblasts ( Fig. 7d ). Moreover, overexpression of ProT in 293T cells upregulated the mRNA expression of MMP2 and MMP9 ( Fig. 7e ). Analysis of microarray data from the lung tissues of smokers with severe emphysema from GEO [20] also revealed a positive correlation between the expression levels of ProT and those of MMP2, as well as between the expression levels of ProT and those of MMP9 ( Supplementary Fig. S5 ). Furthermore, immunohistochemical staining demonstrated that the expression of MMP9 was higher in the lungs of ProT transgenic mice and that CSE treatment upregulated MMP9 expression in both ProT transgenic and NT mice ( Fig. 7f ). Conversely, lentivirus-mediated knockdown of endogenous ProT in the lungs of wild-type FVB mice reduced the expression of MMP9, as compared with the control mice that received Luc shRNA, in CSE-induced emphysema ( Fig. 7g ). Collectively, these results indicate that ProT has a role in the regulation of NF-κB-dependent MMP2 and MMP9 production in the pathogenesis of emphysema. 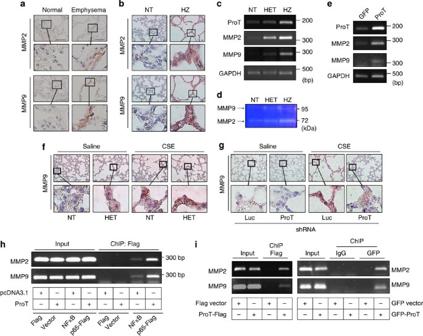Figure 7: ProT upregulates the production of MMP2 and MMP9 in emphysematous lungs of mice and patients. (a,b) Immunohistochemical detection of MMP2 and MMP9 in lung tissues from patients with emphysema and non-COPD individuals (Scale bar=100 μm) (a) and from ProT HET and NT mice (Scale bar=20 μm) (b). (c,e) Expression of MMP2, MMP9, ProT and GAPDH (serving as the loading control) mRNA in lung tissues of 4-day-old ProT HZ, HET and NT mice (c) and in 293 T cells transduced with lentiviral vectors Lenti-ProT or Lenti-GFP (e), as analysed by RT–PCR. (d) Gelatin zymography of MMP2 and MMP9 in the conditioned medium of mouse embryonic fibroblasts (MEF) from ProT transgenic and NT mice. (f,g) Immunohistochemical detection of MMP9 in lung tissues (Scale bar=20 μm) from ProT HET and NT mice injected intraperitoneally with CSE or saline twice a week for 6 weeks (f) and from FVB mice that had been intratracheally injected with lentiviral vectors expressing ProT or luciferase (Luc) shRNA followed by intraperitoneal injections of CSE or saline twice a week for 6 weeks (g). The boxed areas in upper panels (× 400) are magnified and shown in lower panels (a,b,f,g). (h) ChIP analysis showing increases in NF-κB binding toMMP2andMMP9promoters by ProT overexpression. 293T cells that had been transfected with pcDNA3.1-ProT-myc/His or pcDNA3.1 were cotransfected with Flag-tagged NF-κB p65 expression vector or a control vector. Cross-linked chromatin was immunoprecipitated with anti-Flag-M2 beads and then amplified for theMMP2orMMP9gene region containing the NF-κB binding site. Cell lysates without immunoprecipitation (input) were estimated for chromatin containingMMP2orMMP9gene region. (i) ChIP analysis showing direct binding of ProT to the NF-κB-binding site-containing region ofMMP2andMMP9promoters. 293T cells were transfected with plasmid Flag-tagged ProT (pCMV-Tag4A-ProT) or Flag control vector (left) or GFP-tagged ProT or GFP alone (right). Cross-linked chromatin was immunoprecipitated with anti-Flag-M2 beads (left) or anti-GFP or anti-IgG antibody combined with protein A plus G sepharose (right) followed by amplification of theMMP2orMMP9gene region containing NF-κB binding sites. Results are representative of three independent experiments. Figure 7: ProT upregulates the production of MMP2 and MMP9 in emphysematous lungs of mice and patients. ( a , b ) Immunohistochemical detection of MMP2 and MMP9 in lung tissues from patients with emphysema and non-COPD individuals (Scale bar=100 μm) ( a ) and from ProT HET and NT mice (Scale bar=20 μm) ( b ). ( c , e ) Expression of MMP2, MMP9, ProT and GAPDH (serving as the loading control) mRNA in lung tissues of 4-day-old ProT HZ, HET and NT mice ( c ) and in 293 T cells transduced with lentiviral vectors Lenti-ProT or Lenti-GFP ( e ), as analysed by RT–PCR. ( d ) Gelatin zymography of MMP2 and MMP9 in the conditioned medium of mouse embryonic fibroblasts (MEF) from ProT transgenic and NT mice. ( f , g ) Immunohistochemical detection of MMP9 in lung tissues (Scale bar=20 μm) from ProT HET and NT mice injected intraperitoneally with CSE or saline twice a week for 6 weeks ( f ) and from FVB mice that had been intratracheally injected with lentiviral vectors expressing ProT or luciferase (Luc) shRNA followed by intraperitoneal injections of CSE or saline twice a week for 6 weeks ( g ). The boxed areas in upper panels (× 400) are magnified and shown in lower panels ( a , b , f , g ). ( h ) ChIP analysis showing increases in NF-κB binding to MMP2 and MMP9 promoters by ProT overexpression. 293T cells that had been transfected with pcDNA3.1-ProT-myc/His or pcDNA3.1 were cotransfected with Flag-tagged NF-κB p65 expression vector or a control vector. Cross-linked chromatin was immunoprecipitated with anti-Flag-M2 beads and then amplified for the MMP2 or MMP9 gene region containing the NF-κB binding site. Cell lysates without immunoprecipitation (input) were estimated for chromatin containing MMP2 or MMP9 gene region. ( i ) ChIP analysis showing direct binding of ProT to the NF-κB-binding site-containing region of MMP2 and MMP9 promoters. 293T cells were transfected with plasmid Flag-tagged ProT (pCMV-Tag4A-ProT) or Flag control vector (left) or GFP-tagged ProT or GFP alone (right). Cross-linked chromatin was immunoprecipitated with anti-Flag-M2 beads (left) or anti-GFP or anti-IgG antibody combined with protein A plus G sepharose (right) followed by amplification of the MMP2 or MMP9 gene region containing NF-κB binding sites. Results are representative of three independent experiments. Full size image We further investigated whether NF-κB-binding sites were involved in ProT-induced MMP2 and MMP9 expression. A chromatin immunoprecipitation (ChIP) assay revealed that overexpression of ProT increased the binding of NF-κB to the MMP2 and MMP9 promoters ( Fig. 7h ). Furthermore, ProT could directly bind to the NF-κB binding site-containing region within MMP2 and MMP9 promoters ( Fig. 7i ). These findings demonstrate the functional importance of ProT-induced binding of NF-κB to MMP2 and MMP9 promoters. Our data suggest that ProT can occupy NF-κB-dependent promoters and directly increase NF-κB acetylation, thereby enhancing the transcriptional activation of NF-κB on MMP2 and MMP9 promoters. Taken together, our results demonstrate that overexpressed ProT associates with MMP2 and MMP9 promoters and results in increased levels of acetylated NF-κB at the promoters, which is associated with CS-mediated production of MMP2 and MMP9. CS is the main risk factor for emphysema, acting through the acetylation-mediated enhancement of chromatin remodelling in pro-inflammatory genes [2] , [31] . However, other factors, including genetic or host factors, may also be important in the development of emphysema. We tested the hypothesis that ProT regulates acetylation events and hence has a critical role in predisposing individuals to develop emphysema. In this study, we demonstrated for the first time the correlation between ProT and emphysema in both clinical patients and ProT transgenic mice. Our results indicate that overexpression of ProT in the lung is correlated with severity of emphysema in clinical patients. In animal models, ProT HZ transgenic mice exhibited spontaneous airspace enlargement and alveolar wall destruction, which are characteristics of emphysema. The HET mice had only mild airspace enlargements; however, treatment with CSE significantly increased the incidence and severity of emphysema with concomitant enhancements in ProT expression. We also showed that the increase in airspace enlargement was associated with elevated levels of acetylated NF-κB (p65 Lys310) that colocalized with ProT in the nucleus and with increased MMP2 and MMP9 levels in the lungs of ProT transgenic mice. More significantly, our RNA interference experiments verified that endogenous ProT affects NF-κB acetylation and MMP production in the development of emphysema, especially upon exposure to CS. These results clearly indicate the clinical relevance of ProT in the development of pulmonary emphysema. The balance between protein acetylation and deacetylation that maintains cellular homeostasis is determined by the HAT/HDAC interplay. Previous studies have demonstrated that ProT is involved in chromatin remodelling by binding to histones as well as by recruiting and stabilizing HAT CBP/p300 coactivators, thus regulating gene transcription [12] , [14] , [16] , [17] . In this study, we further demonstrated that in addition to histones, ProT has a role in the post-translational acetylation of non-histone proteins, including NF-κB (p65 Lys310) involved in regulating the expression of pro-inflammatory genes in COPD. Moreover, we observed decreases in HDAC2 levels, which correlated with disease severity, but no detectable changes in HDAC1 and HDAC3 proteins in the lungs of emphysema patients or ProT transgenic mice. These results are consistent with a previous report showing a marked reduction in the HDAC2 expression in the lungs of COPD patients [22] . Surprisingly, we also found that ProT is capable of inhibiting the interaction of HDAC2 or HDAC1 with histones. Furthermore, ProT can directly bind to NF-κB and enhance its acetylation by displacing HDAC3 from its complex with NF-κB. As HDAC1 and HDAC2 can also interact with RelA/p65 and inhibit its transactivation [32] , ProT also probably affects these two HDACs through the same mechanism. We demonstrated for the first time that ProT can inhibit class I HDACs, including HDAC1, 2 and 3, and thereby enhance the acetylation of histones and NF-κB. Our results from animal models and clinical patients strongly suggest a potential novel model whereby excess ProT causes a shift in the HAT/HDAC balance toward HAT in the emphysematous lung, which supports an important role for ProT in the pathogenesis of emphysema. We propose that the mechanisms of ProT action in combination with CS exposure in emphysema underlie the hyperacetylation of chromatin and NF-κB, leading to upregulation of NF-κB-dependent gene expression, such as MMP2 and MMP9 ( Fig. 8 ). Reduction of other deacetylases, such as SIRT1, has been found in macrophages and in the lungs of smokers and COPD patients, and it leads to increased acetylation and activation of p65 (ref. 33 ). As many proteins are subject to lysine acetylation, which can modulate protein interaction, DNA binding and subcellular localization, it is tempting to speculate that ProT may affect their functions through the regulation of the HAT/HDAC balance. It is conceivable that, in addition to the acetylation of the histones and NF-κB that regulate these inflammatory responses, other unidentified molecules and pathways are also affected by overexpressed ProT and contribute to the pathogenesis of emphysema. 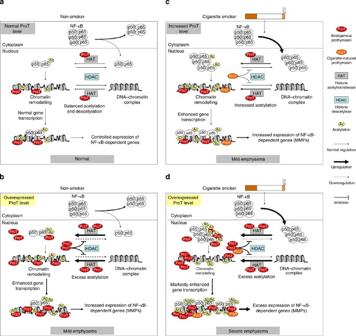Figure 8: Proposed model for the regulation of HAT/HDAC by ProT in emphysema. (a) Healthy individuals who do not smoke cigarettes maintain the HAT/HDAC balance and thereby sustain normal transcription of NF-κB-dependent genes. (b) Non-smokers who have higher basal ProT levels exhibit reduced association of HDACs with histones in the lung. This leads to enhancing acetylation-mediated chromatin remodelling and thereby upregulating the expression of NF-κB-dependent genes, such asMMP2andMMP9. Thus, such individuals may develop mild emphysema. (c) In smokers who have normal ProT basal levels, exposure to CS induces ProT expression and nuclear translocation of NF-κB in the lung. This results in reduced HDAC activity and increased acetylation of chromatin and NF-κB, and in turn leads to upregulation of the transcription of NF-κB-dependent genes, such asMMP2andMMP9. This ultimately causes emphysema. Long-term cigarette smoking may exacerbate this effect and increase the severity of emphysema. (d) In smokers who have higher basal ProT levels, CS exposure further upregulates ProT expression. Excess ProT causes a shift in the HAT/HDAC balance toward HAT. This results in developing severe emphysema. Thus, ProT predisposes individuals to CS-induced emphysema. Figure 8: Proposed model for the regulation of HAT/HDAC by ProT in emphysema. ( a ) Healthy individuals who do not smoke cigarettes maintain the HAT/HDAC balance and thereby sustain normal transcription of NF-κB-dependent genes. ( b ) Non-smokers who have higher basal ProT levels exhibit reduced association of HDACs with histones in the lung. This leads to enhancing acetylation-mediated chromatin remodelling and thereby upregulating the expression of NF-κB-dependent genes, such as MMP2 and MMP9 . Thus, such individuals may develop mild emphysema. ( c ) In smokers who have normal ProT basal levels, exposure to CS induces ProT expression and nuclear translocation of NF-κB in the lung. This results in reduced HDAC activity and increased acetylation of chromatin and NF-κB, and in turn leads to upregulation of the transcription of NF-κB-dependent genes, such as MMP2 and MMP9 . This ultimately causes emphysema. Long-term cigarette smoking may exacerbate this effect and increase the severity of emphysema. ( d ) In smokers who have higher basal ProT levels, CS exposure further upregulates ProT expression. Excess ProT causes a shift in the HAT/HDAC balance toward HAT. This results in developing severe emphysema. Thus, ProT predisposes individuals to CS-induced emphysema. Full size image NF-κB is involved in many pathways, including inflammation, cell survival, proliferation and differentiation. The typical NF-κB pathway is characterized by activation of p50/p65 heterodimers to transactivate pro-inflammatory gene expression [34] . Homodimers of the p50 subunit, which lack transactivation domains, can repress NF-κB target gene expression. Gene knockout studies have shown that NF-κB can have both pro-inflammatory and anti-inflammatory roles that are probably involved in the resolution of inflammation [35] . The p65 knockout mice were embryonically lethal; however, p50 knockout mice that are HET for p65 were more susceptible to lipopolysaccharide-induced shock, suggesting an anti-inflammatory role for p50/p65 heterodimers [36] . Interestingly, p50-null mice with normal p65 genes showed spontaneous airspace enlargement with concomitant increases in the phosphorylation, acetylation (Lys310) and DNA-binding activity of p65 in the lung, which were further increased after CS exposure [37] . These animal studies indicate the importance of the transactivation function of acetylated p65 for the pro-inflammatory activity of NF-κB. In line with this notion, our results indicate that ProT has an important role in the acetylation and activation of NF-κB, particularly upon CS exposure, within the pathogenesis of emphysema. Nevertheless, the clinical significance of the anti-inflammatory role of NF-κB in emphysema has yet to be established. Besides inflammation, oxidative stress also has an important role in CS-mediated emphysema. Nrf2 is a nuclear transcription factor that controls the expression and coordinated induction of defensive genes encoding detoxifying enzymes and antioxidant proteins. Nrf2 knockout mice exhibited enhanced susceptibility to CS-induced emphysema [38] . ProT can regulate the Nrf2-Keap1 (inhibitor of Nrf2, also known as INrf2) system, suggesting that it has a role in oxidative stress defense [39] , [40] . ProT can dissociate the Nrf2–Keap1 complex by interaction with Keap1, thus upregulating the expression of Nrf2-dependent oxidative stress-protecting genes [39] . A seemingly conflicting report showed that ProT can mediate the nuclear import of the INrf2/Cul3 Rbx1 complex to degrade nuclear Nrf2 and rapidly switch off the activation of Nrf2 downstream gene expression [40] . These studies suggest the potential involvement of ProT in the on/off switch of Nrf2-Keap1 mechanisms. Furthermore, NF-κB can antagonize the Nrf2-antioxidant response element pathway by both depriving CBP from Nrf2 and promoting the recruitment of HDACs to antioxidant response element, suggesting a possible role for NF-κB in suppressing the expression of anti-inflammatory genes [41] . However, the clinical relevance of the interplay between ProT and NF-κB in the Nrf2–Keap1 system remains to be determined. Whether overexpressed ProT in the lungs of patients or mice with emphysema effects the expression of Nrf2-dependent genes, particularly in response to CS, requires further investigation. ProT may exert differential effects depending on its cellular localization. It not only functions in the nucleus as described here, but also has a significant anti-apoptotic role in the cytoplasm by binding to cytochrome c and hence inhibiting cytochrome c -induced caspase activation and apoptosis [42] , [43] , as well as by directly inhibiting the apoptosome, an important complex in the execution of apoptosis [44] . Additionally, extracellular ProT has a neuroprotective role in cerebral ischemia-induced damage [45] , [46] . The cytoprotective function of ProT appears to be in opposition to our results, demonstrating the involvement of ProT in oxidative stress-induced lung tissue injury, a mechanism that contributes to the pathogenesis of CS-mediated emphysema. We show that ProT is overexpressed in the nucleus of emphysematous tissues from clinical patients and ProT transgenic mice and in a mouse model of CS-induced emphysema. The nuclear role of ProT is more closely related than its cytoplasmic or extracellular role to the elevation of acetylated chromatin and NF-κB transactivation found in the emphysematous lung, further supporting the clinical relevance of ProT in terms of emphysema pathogenesis. Our results from patients with emphysema and animal models indicate that excess ProT in the lung contributes to the development of emphysema and that CS exposure exacerbates disease severity by further promoting ProT expression. Our data reveal a novel function of ProT of inhibiting HDAC expression and activity. We also provide evidence linking ProT with NF-κB in emphysema. Our findings may further illuminate how CS mediates the chromatin remodelling of pro-inflammatory genes and reduction of HDAC activity in the development of emphysema. As COPD is poorly responsive to the anti-inflammatory actions of corticosteroids due to reduced HDAC activity [2] , [47] , [48] , ProT may serve as a novel therapeutic target to overcome this major therapeutic barrier. Oxidative stress triggered by components of CS can induce ERK-dependent phosphorylation of c-myc, hence promoting the stability and accumulation of c-myc [49] , [50] . As ProT is a target gene of c-myc [51] , it is tempting to postulate that CS-induced ProT overexpression in emphysema may be attributable, in part, to the activation of c-myc. Further studies are required to elucidate the mechanism of CS-mediated upregulation of ProT in the pathogenesis of emphysema. Clinical samples and mice Clinical samples were collected from 20 patients with a diagnosis of emphysema who underwent surgery at the Thoracic Division, Department of Surgery, National Cheng Kung University (NCKU) Hospital. Among them, eight patients with severe to very severe emphysema underwent lung volume reduction surgery or lung transplantation, and the remainder with mild-to-moderate emphysema received a bullectomy or wedge resection for the treatment of pneumothorax. The severity of emphysema was spirometrically classified according to the criteria of the Global initiative for chronic obstructive lung disease. Eight of twelve patients with mild or moderate emphysema and seven of eight patients with severe and very severe emphysema were smokers. The clinical characteristics of COPD patients are summarized in Supplementary Table S1 . The samples that served as ‘normal’ controls were from the non-tumour parts of the resected lobes of four patients who were cigarette smokers without COPD and who had undergone surgery for lung cancer. Informed consent was obtained from all subjects, and the experimental protocol was approved by the Human Experiment and Ethics Committee, NCKU Hospital. ProT transgenic mice were generated and screened as described previously [19] . The experimental protocol adhered to the rules of the Animal Protection Act of Taiwan and was approved by the Laboratory Animal Care and Use Committee of NCKU. Cells and plasmids Human A549 lung adenocarcinoma cells and murine MLE 12 lung epithelial cells were originally obtained from American Type Culture Collection (ATCC). Human 293T embryonic kidney cells were obtained from the National RNAi Core Facility, Academia Sinica, Taiwan. The commercially available plasmids that were used in this study included pCMVb p300 HA delta33, which encodes human p300 mutant protein lacking amino acids 1737–1836; pcDNA3.1-HDAC1-Flag; pcDNA3.1-HDAC3-Flag; and pcDNA3-cFlag-RelA, each of which was purchased from Addgene; as well as pHM6-lacZ (Roche), pNF-κB-Luc (Clontech), pTK-Renilla (Promega) and pCMV-Tag2B (Stratagen). The plasmids used in this study were constructed as follows. The cDNA fragment of mouse ProT was excised from pJ6Ω-ProT [19] by digestion with Hin dIII and Eco RI and then cloned into the Hin dIII/ Eco RI sites of pcDNA3.1 and pcDNA3.1/myc-His (Invitrogen) to generate pcDNA3.1-ProT and pcDNA3.1/ProT-myc/His, respectively. Subsequently, pcDNA3.1-ProT was digested with Pme I and Eco RI to excise the ProT coding sequence, which was then ligated into the Pme I/ Eco RI sites of pWPXL [52] to replace the GFP gene to yield pWPXL-ProT. An IRES-GFP fragment was excised from PWPI by Eco RI digestion and subcloned into the Eco RI site of pWPXL-ProT to generate pWPXL-ProT-IRES-GFP. The pcDNA3.1-ProT was digested with Hin dIII and Pme I and subcloned into the the Hin dIII/ Sma I sites of pEGFP-C1 (Clontech) to generate a GFP-tagged ProT expression plasmid (pEGFP-C1-ProT). Moreover, the CMV promoter-driven Flag-tagged fusion cassette was excised from pCMV-tag2B by Nde I and Bam HI digestion and cloned into the Nde I/ Bgl II sites of pEGFP-C1-ProT to replace the GFP coding sequence, yielding a Flag-tagged ProT expression plasmid (pCMV-tag2B-ProT). The cDNA fragment (1,591 bp) of human HDAC2 was obtained from the reverse transcriptase-polymerase chain reaction (RT–PCR) amplification of mRNA from 293T cells with forward primer 5′-ACTATCGCCCCCAC GGATCC CTCA-3′ and the reverse primer 5′-TTTC CAATTG AGGGGTTGCTGAGCTGTTCTG-3′ in which a Bam HI site and an Mfe I site (underlined) were introduced onto the 5′-end and the 3′-end, respectively. The resulting PCR amplicons were digested with Bam HI and Mfe I and subcloned into the Bam HI/ Eco RI sites of pCMV-tag4C (Stratagen) to generate a Flag-tagged HDAC2 expression plasmid (pCMV-tag4C-HDAC2). Lentiviral vectors Recombinant lentiviruses coexpressing ProT and enhanced green fluorescent protein (EGFP) or expressing either EGFP-tagged ProT or EGFP alone were individually produced by the transient transfection of 293T cells with pWPXL-ProT-IRES-GFP, pWPXL-EGFP-ProT and pWPT, along with the packaging construct psPAX2 and the VSV-G expression plasmid pMD2G [53] . For the ProT knockdown experiments, pLKO.1-puro-based lentiviral vectors including stem-loop cassettes encoding shRNA for human ProT (TRCN0000138110, 0000135421, 0000133816, 0000134223 and 0000138750; designated ProT shRNA-1–5), mouse ProT (TRCN0000125359, 0000125360, 0000125361, 0000125362 and 0000125363; designated ProT shRNA 12–15) and luciferase (TRCN 0000072246; designated Luc shRNA) were used. On the basis of real-time RT–PCR analysis, the most efficient shRNA for knockdown of human ProT (shRNA-2) or mouse ProT (shRNA 15) was selected for lentiviral production. Lentiviruses were produced and titrated as previously described [52] . CSE and animal models The CSE was prepared as described with slight modifications [21] , [22] , [54] . One cigarette (Marlboro, Philip Morris USA Inc.) was burned, and the smoke was imported to a vessel containing saline (3 ml per cigarette) using a vacuum pump. The CSE-saline solution was freshly prepared and sterilized via filtration through a 0.22-μm Millipore filter for each injection. Six-week-old male FVB mice or ProT HET transgenic mice were injected intraperitoneally with 0.5 ml of CSE-saline or saline twice a week for 6 weeks. The mice were killed, and the lung tissue sections were subjected to H&E staining and examined for alveolar airspace enlargement. Average airspace area was calculated by dividing the total airspace by the total number of alveoli using MetaMorph software (Universal Imaging Corp.) [55] . For the in vivo knockdown experiments, six-week-old FVB mice were intratracheally injected with lentiviral vectors expressing shRNA specific to ProT or Luc followed by intraperitoneal injections of CSE or saline twice a week for 6 weeks. Immunological assays For the immunohistochemical studies, 5-μm-thick sections of paraffin-embedded human or mouse lung tissue blocks were prepared. The primary antibodies used included monoclonal antibodies against ProT (clone 2F11, ascites fluid) [56] , [57] and polyclonal antibodies against HDAC1 (1:100, Santa Cruz), HDAC2 (1:100, Santa Cruz), HDAC3 (1:100, Santa Cruz), acetylated-lysine (1:800, Cell Signaling), acetylated-Lys310 NF-κB p65 (1:100, Genetex), MMP2 (1:50, Santa Cruz) and MMP9 (1:50, Santa Cruz). Tissue sections were incubated with primary antibodies at 4 °C overnight followed by incubation with horseradish peroxidase-conjugated goat anti-mouse, goat anti-rabbit or donkey anti-goat IgG (1:200, Jackson) at room temperature for 2 h. Negative controls included sections stained with mouse universal negative control (Dako) and isotype control IgG (Santa Cruz). The reactivity was visualized with aminoethyl carbazole (red colour, Zymed) and counterstained with hematoxylin. Immunoblotting and immunoprecipitation were performed using standard methods. As ProT is a highly acidic protein and is poorly retarded by the nitrocellulose membrane at standard electrotransfer conditions, protein samples were transferred by an acidic transfer method onto a PVDF membrane (Millipore) to immobilize ProT [57] . The primary antibodies used for immunoblotting included antibodies against ProT (clone 2F11), acetylated-lysine (1:1000, Cell Signaling), HDAC1 (1:1000, Santa Cruz), HDAC2 (1:1000, Santa Cruz), HDAC3 (1:1000, Santa Cruz), histone H1 (1:2000, Santa Cruz), acetylated-histone H1 (1:1000, Genetex), histone H3 (1:2000, Santa Cruz), acetylated-histone H3 (1:1000, Cell Signaling), NF-κB p65 (1:1000, Santa Cruz), acetylated-Lys310 NF-κB p65 (1:1000, Genetex), p300 (1:500, Santa Cruz) and β-actin (1:10,000, Abcam). horseradish peroxidase-conjugated goat anti-mouse, goat anti-rabbit or donkey anti-goat IgG (Jackson) were used as secondary antibodies where appropriate, and protein–antibody complexes were detected by the ECL system (Millipore) and visualized with a Biospectrum AC imaging system (UVP). Images of full-length blots are shown in Supplementary Fig. S6 . For immunofluorescence, the cells were incubated with ProT (clone 2F11) and acetylated-lysine (1:800, Cell Signaling) antibodies and subsequently incubated with Alexa Fluor 594-conjugated goat anti-mouse IgG (Invitrogen) and FITC-conjugated goat anti-rabbit IgG (KPL). The nuclei were counterstained with DAPI (Sigma-Aldrich). Fluorescence signals were examined by fluorescence microscopy. RT–PCR analysis Total RNA was isolated from the lung tissue of transgenic mice or lentivirus-transduced cells using QuickGene RNA tissue or a cultured cell kit (Fujifilm), and 2 μg of RNA was used for cDNA synthesis using a reverse iT first-strand synthesis kit (Thermo) according to the manufacturer’s instructions. The following primers were used for RT–PCR: human and mouse ProT, 5′-AAGGAGAAGAAGGAAGTTGTGGA-3′ (forward) and 5′-CTACCTCATTGTCAGCCTCCTG-3′ (reverse); mouse MMP2, 5′-GAGGATACCCCAAGCCACTGA-3′ (forward) and 5′-CCAGCCAGTCTGATTTGATGCT-3′ (reverse); mouse MMP9, 5′-TAAAACGCAGCTCAGTAACAGTCCG-3′ (forward) and 5′-TGGAATCCTGTGGCATCCATGAAAC-3′ (reverse); human MMP2, 5′-CTGGAGATACAATGAGGTGAAGAAG-3′ (forward) and 5′-AAGGCAGTGGAGAGGAAGGG-3′ (reverse); human MMP9, 5′-GCATAAGGACGACGTGAATGGC-3′ (forward) and 5′-GGACTCAAAGGCACAGTAGTGG-3′ (reverse); human and mouse GAPDH, 5′-ACTTCAACAGCGACACCCACT-3′ (forward) and 5′-GCCAAATTCGTTGTCATACCAG-3′ (reverse). The PCR products were separated by 1% agarose gel electrophoresis. ChIP assay ChIP was performed using the EZ-CHIP kit (Millipore). Briefly, the proteins were formaldehyde (1%) crossed-linked to chromatin in 293T cells that had been transfected with Flag- or GFP-tagged ProT or with Flag-tagged NF-κB p65 plasmid DNA. The cell lysates were sonicated with alternating 30 s pulses 10 times by a sonicator (Microson XL2000, Misonix Inc., Farmingdale, NY, USA) to shear DNA to lengths between 500 and 1,000 bp followed by immunoprecipitation with anti-Flag-M2 beads (Sigma-Aldrich), or with anti-GFP (Santa Cruz) or anti-IgG (Santa Cruz) antibodies in combination with protein A plus G sepharose (Santa Cruz). The immunoprecipitates were washed and reverse cross-linked. PCR was performed on the phenol–chloroform-extracted DNA to detect the NF-κB-binding sites within the MMP2 and MMP9 promoters with specific primers as described previously [58] , [59] . The PCR primers used in ChIP included MMP2, 5′-GGTTCCAACGTCTCTAACG-3′ (forward) and 5′-CAGATGATCAGCCACAATG-3′ (reverse); MMP9, 5′- AGTGGTAAGACATTTGCCCGA-3′ (forward) and 5′-TGCAACACCCCCTCCCAGGTCAG-3′ (reverse). The PCR products were separated by 1% agarose gel electrophoresis. Zymography The enzymatic activities of MMP2 and MMP9 were determined by gelatin zymography as previously described [60] . The conditioned medium collected from the mouse embryonic fibroblasts of ProT transgenic or NT mice was electrophoresed on 10% SDS–PAGE gels containing 1 mg ml −1 gelatin (Sigma-Aldrich) to assess MMP2 and MMP9 activity. Statistical analysis Statistical analyses were performed using SigmaStat 3.5 (Systat Software). Statistical significance was assessed with Student’s t- test. Correlations were measured using Pearson’s correlation coefficient ( r ). How to cite this article: Su, B.-H. et al . Prothymosin α overexpression contributes to the development of pulmonary emphysema. Nat. Commun. 4:1906 doi: 10.1038/ncomms2906 (2013).